Free energy landscape of activation in a signalling protein at atomic resolution The interconversion between inactive and active protein states, traditionally described by two static structures, is at the heart of signalling. However, how folded states interconvert is largely unknown due to the inability to experimentally observe transition pathways. Here we explore the free energy landscape of the bacterial response regulator NtrC by combining computation and nuclear magnetic resonance, and discover unexpected features underlying efficient signalling. We find that functional states are defined purely in kinetic and not structural terms. The need of a well-defined conformer, crucial to the active state, is absent in the inactive state, which comprises a heterogeneous collection of conformers. The transition between active and inactive states occurs through multiple pathways, facilitated by a number of nonnative transient hydrogen bonds, thus lowering the transition barrier through both entropic and enthalpic contributions. These findings may represent general features for functional conformational transitions within the folded state. Studies on the interconnection between protein structure, dynamics and function have delineated a paradigm describing the folded state of proteins as composed by well-defined conformations, often structurally characterized by nuclear magnetic resonance (NMR) or X-ray crystallography, corresponding to different functional states [1] . The crucial role of ‘protein dynamics’ for biological function, describing the ability of interconverting between these specific conformers, has recently gained increased attention in structural biology. Changing conformation allows proteins to catalyze chemical reactions or control the response to environmental stimuli. While significant progress has been made in the structural characterization of the conformers, the understanding of how folded proteins can efficiently interconvert between the functional important states while avoiding detrimental unfolding is in its infancy. This is reflected in the poor performance of designed enzymes relative to naturally evolved ones, since current designs are aimed at one specific conformation based on the predicted transition state structure [2] , [3] . The question of ‘how’ proteins interconvert is a question of pathways. Due to recent impressive computational developments, pathways of conformational transitions within the folded state have been directly observed for a few proteins in unbiased molecular dynamics (MD) simulations [4] , [5] , [6] , [7] , [8] , [9] , [10] . Here we investigate the full free energy landscape of the inactive/active interconversion of the receiver domain of Nitrogen Regulatory Protein C (NtrC R ), resulting in unexpected findings of new principles defining native state energy landscapes. NtrC R , a response regulator of a bacterial two-component system that, upon phosphorylation by its cognate histidine kinase NtrB, activates the transcription of genes in response to nitrogen starvation, has been instrumental for studying functional conformational changes. A body of experimental data is available [11] , [12] , [13] , [14] . NtrC R exists in its apo form in a mixed equilibrium of its active and inactive states, with an interconversion rate of ∼ 13,000 s −1 (refs 11 , 12 , 13 ). This equilibrium is shifted on phosphorylation of aspartate 54 via stabilization of the active state [13] , which promotes the propagation of the signal to the downstream partners [13] , [15] . Details of the global inactive–active conformational change ( Fig. 1a ) [11] , [12] , [14] have been investigated by experiments, followed by computational methods using simplified coarse grained models [16] , [17] , [18] , [19] and full atomistic MD simulations [20] , [21] , [22] , [23] . Very different transition pathways have been proposed, ranging from transitions via a partial unfolding of the helix [17] , to mechanisms in which helix α4 remains stable throughout the transition [22] . Many studies on NtrC R and other homologous response regulators have focused on the interaction between the conserved Y101 and T82. This interaction (dubbed ‘T-Y coupling’) had been suggested to be crucial in triggering the inactive–active conformational transition [24] , but has recently been shown to not be necessary for the activation process [25] , illustrating the controversial views of the mechanism of signal activation in this protein family. 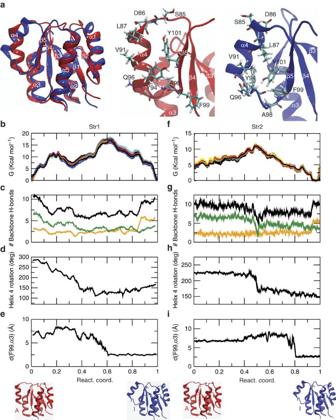Figure 1: Free energy landscape of active/inactive transition of NtrCRexplored by the string method. (a) Inactive (blue) and active (red) models of NtrCRare overlaid11and a zoom-in is shown highlighting the difference in conformation concentrated in the area of helix 4. The conformational change involves a different span of the helix in the sequence, a change in helix orientation, a rotation around the helical axis and a rearrangement of sidechains, including Y94, Q96 and Y101. (b) Estimated free energy profile along the pathway for string 1; different profiles have been estimated repeating the weighted histogram analysis 10 times (shown in different colours), removing each time 10–20% of the data to provide an estimation of the uncertainties, (c) number of backbone H-bonds in helix 4 (black) and in the lower (residues 90–96, green) and upper part (residues 84–90, yellow) of helix 4, (d) rotation of helix 4 around its axis and (e) minimum distance of the sidechain of F99 from helix 3. (f–i) Similar plots for the string Str2. Figure 1: Free energy landscape of active/inactive transition of NtrC R explored by the string method. ( a ) Inactive (blue) and active (red) models of NtrC R are overlaid [11] and a zoom-in is shown highlighting the difference in conformation concentrated in the area of helix 4. The conformational change involves a different span of the helix in the sequence, a change in helix orientation, a rotation around the helical axis and a rearrangement of sidechains, including Y94, Q96 and Y101. ( b ) Estimated free energy profile along the pathway for string 1; different profiles have been estimated repeating the weighted histogram analysis 10 times (shown in different colours), removing each time 10–20% of the data to provide an estimation of the uncertainties, ( c ) number of backbone H-bonds in helix 4 (black) and in the lower (residues 90–96, green) and upper part (residues 84–90, yellow) of helix 4, ( d ) rotation of helix 4 around its axis and ( e ) minimum distance of the sidechain of F99 from helix 3. ( f – i ) Similar plots for the string Str2. Full size image Here by combining multiple computational enhanced sampling methods with new NMR data, we demonstrate that the free energy landscape is significantly more complex than described previously, transgressing the boundaries of the general paradigm that the active and inactive states are constituted by two well-defined structures. We show that the inactive state cannot be described by a single structure, but rather by an ensemble of structurally different conformers with comparable free energy. In contrast, the conformers belonging to the active state ensemble are much more structurally homogeneous. Consequently, NtrC R ’s functional states do not correspond to two precise conformations, but rather have to be defined kinetically. Strikingly, the interconversion between the active and inactive ensembles occurs via multiple transition pathways engaging a number of nonnative H-bonds, which results in both an entropic and enthalpic lowering of the energy barrier. Free energy profiles display the landscape complexity We started our investigation based on the generally accepted paradigm of interconversion between the well-defined inactive and active structures. The differences between the active and inactive NMR structures were concentrated in the region of helix α4, allosterically communicating with the phosphorylation site D54 (refs 12 , 13 , 14 ; Fig. 1a ). The NMR structures together with targeted MD simulations (TMD) [13] , [22] suggested that the system interconverts between these two well-defined conformations [13] . To obtain quantitative energetic information on the atomistic details of the conformational transition, and alleviate potential artifacts introduced by the biased simulations in the previous TMD study conducted by some of us [13] , [22] , we applied here a pathway calculation method, the string method, in the implementation proposed by Pan et al. [18] . The TMD trajectory, used as initial trajectory, was progressively relaxed in the multidimensional space of relevant collective variables towards the local minimum free energy pathway. The free energy profile was estimated using umbrella sampling along the arc-length measured on the final relaxed pathway ( Fig. 1b,f ). The calculation was repeated two times, using two independently generated TMDs as initial pathway ( Supplementary Fig. 1 ). While both strings (Str1 and Str2) undergo analogous steps along the transition, the two pathways did not converge to one ( Fig. 1b–i , Supplementary Fig. 1 ), but maintain qualitative differences similar to those observed in the original TMD trajectories. In other systems it has been reported that the string method converged to the same final trajectory from different initial ones [26] . Our result may be an indication that the conformational landscape of NtrC R is extremely corrugated, with different available pathways separated by significant barriers which cannot be overcome by the short sampling performed during the pathway optimization procedure. The two free energy profiles ( Fig. 1b,f ) present important common traits, for instance that the profiles are dominated by a single main barrier. The free energy profiles identify the various events occurring during the transitions, captured by relevant order parameters plotted in Fig. 1c–e and g–i . In both Str1 and Str2, the loss of helical content in the C terminus of helix 4 (green curve in Fig. 1c,g ) appears correlated to the change in the rotation around the helix axis ( Fig. 1d,h ). This event represents the rate-limiting step in the transition described by Str2, while in Str1 the main barrier is related to the rearrangement of the loop connecting α4 and β5. In the model of the inactive state ( Fig. 1a ), the sidechains of F99, Y94 and A98 constitute a hydrophobic patch packed against the hydrophobic face of helix α3. In the active state, the positions of Y94 and F99 are switched facing helix α5, whereas Q96, which in the inactive state model was exposed to the solvent, is positioned towards helix α3. This change in hydrophobic packing can be captured by the distance between F99 and helix α3 ( Fig. 1e,i ). In both pathways, the addition of the N-terminal turn of the helix is not directly associated to a major barrier ( Fig. 1c,g ). This analysis of the transition pathways stimulates two crucial questions for understanding the mechanism of activation: what is the relation between the structural rearrangement of the helix 4 backbone and that of the aromatic and hydrophobic sidechains involved in the transition, which need to navigate through a crowded environment? Is the fact that we observe different pathways in our calculations simply due to a sampling limitation in the calculation method we used, or does it reflect an important physical feature of NtrC? The active and inactive states are kinetically defined To address these questions, we used a large number of unbiased MD simulations to build a Markov State Model (MSM), which describes the full conformational landscape bridging the active and inactive conformers. MSMs have been recently applied to represent thermodynamics and kinetic properties of biomolecular systems in the context of protein folding [27] , [28] , [29] , [30] , [31] , [32] , [33] and folded state fluctuations [5] , [6] , [7] , [8] , [9] , [10] , [34] , without the bias of pre-assumed reaction coordinates. Starting from the 80 frames distributed along the pathway Str2, we generated 8,000 simulations using the Folding@home infrastructure [35] , resulting in >1 ms of cumulative simulation time. The lengths of single trajectories varied between a few to several hundreds of nanoseconds ( Supplementary Fig. 2 ). To achieve a comprehensive representation of the free energy landscape from these unbiased MD simulations, we first grouped the complete collection of trajectory snapshots into structurally defined clusters (microstates) according to a structural similarity criterion (see Methods for details). We then used the MD trajectories to estimate the transition probabilities between the identified microstates. A spectral analysis of the transition probability matrix allows the identification of the most relevant slow relaxation processes. The analysis shows one single slow process occurring in about 100 μs ( Supplementary Fig. 2 ). We note that a precise estimate of the slow interconversion rate is not possible due to the limited number of rare transitions sampled. However, this slower process is clearly separated from the rest of the relaxation processes, that represent transitions in the low-microsecond regime and faster, and are consequently better sampled by our simulations. The large separation between the first slow rate and the rest of the transitions suggests that the dynamics of the system can be described within a two-state model as interconversion between two macrostates ( Fig. 2a ). Since the corresponding time scale is comparable to the inactive/active interconversion rate measured experimentally by NMR [13] , the two macrostates in the MSM analysis could in fact represent the two functional active (A) and inactive (I) states. These two macrostates, identified by grouping the 2,168 microstates according to the kinetics using the PCCA procedure [36] , [37] , [38] , have similar populations (about 52 and 48%), but are extremely different in nature. 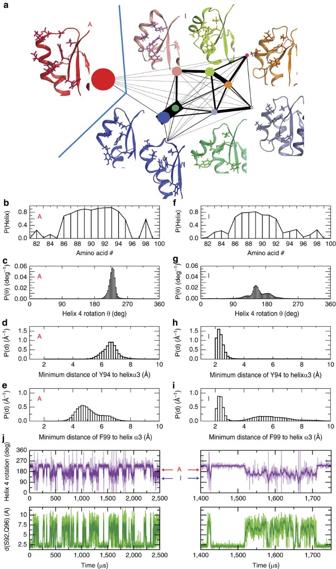Figure 2: Markov State model of active/inactive transition of NtrCR. (a) Force-directed layout of a graph representation of a Markov State model with 10 states. The size of the circles represents the populations of the states and the thickness of connections is proportional to the frequency of transitions among them. Some of the most representative structures in each macrostate are viewed using the same zoom-in used inFig. 1a. The active (A) and inactive (I) state ensembles, which are defined kinetically, are separated by the blue line. (b) The helical propensity for each amino acid is averaged over conformers belonging to the active macrostate. (c) Distribution of values for the rotation of the helix around its axis in the active macrostate, (d,e) distribution of the minimum distances between F99 (d) and Y94 (e) to helix 3 for conformations in the active state. (f–i) Corresponding plots are given for the inactive macrostate. (j) Angle of rotation of the helix 4 (purple) and backbone hydrogen bond distance between S92 and Q96 (green) measured along a meta-trajectory generated with kinetic Monte Carlo sampling on the transition probabilities among the MSM microstates. While the change in the helix rotation marks the transition between the two macrostates, fluctuations in the S92–Q96 distance correspond to transitions among some of the sub-states that constitute the structurally heterogeneous inactive state. The right panels show an expanded view of a portion of the trajectory, highlighting these transitions among inactive sub-states. Figure 2: Markov State model of active/inactive transition of NtrC R . ( a ) Force-directed layout of a graph representation of a Markov State model with 10 states. The size of the circles represents the populations of the states and the thickness of connections is proportional to the frequency of transitions among them. Some of the most representative structures in each macrostate are viewed using the same zoom-in used in Fig. 1a . The active (A) and inactive (I) state ensembles, which are defined kinetically, are separated by the blue line. ( b ) The helical propensity for each amino acid is averaged over conformers belonging to the active macrostate. ( c ) Distribution of values for the rotation of the helix around its axis in the active macrostate, ( d , e ) distribution of the minimum distances between F99 ( d ) and Y94 ( e ) to helix 3 for conformations in the active state. ( f – i ) Corresponding plots are given for the inactive macrostate. ( j ) Angle of rotation of the helix 4 (purple) and backbone hydrogen bond distance between S92 and Q96 (green) measured along a meta-trajectory generated with kinetic Monte Carlo sampling on the transition probabilities among the MSM microstates. While the change in the helix rotation marks the transition between the two macrostates, fluctuations in the S92–Q96 distance correspond to transitions among some of the sub-states that constitute the structurally heterogeneous inactive state. The right panels show an expanded view of a portion of the trajectory, highlighting these transitions among inactive sub-states. Full size image Homogeneous active versus heterogeneous inactive state A more detailed description of the landscape clarifies the distinction between the functional states. When we construct a more detailed MSM, grouping the micro states in 10 macrostates instead of only 2 to explicitly visualize some of the low-microsecond processes, we observe a fragmentation of I into a collection of sub-states, whereas A remains structurally homogeneous ( Fig. 2a shows a graph representation of a MSM with 10 states). The MSM analysis highlights the very heterogeneous nature of I, suggesting that those quite different structures are not simply isolated high-energy states encountered along the pathway towards the active state, but rather represent states with comparable free energies. Only ∼ 5% of the 2,168 microstates are assigned to A. Its structural homogeneity is particularly apparent from the stability of α4 ( Fig. 2b ). Only the loop preceding the N terminus of the helix displays some flexibility. 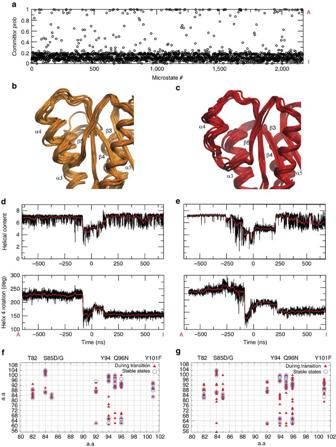Figure 3: Multiple pathways connect the inactive and active states. (a) Committor probabilities for each of the 2,168 microstates in the MSM, defining the 5 most populated microstates belonging to the inactive and active macrostates as reactant and products, respectively. (b,c) Superposition of states with committor probabilities close to 0.5 indicates qualitative differences, ranging from an intact helix 4 (b) to a partially unfolded helix 4 (c). (d,e) Helical content and rotation angle of helix 4 during trajectories describing a full transition between active and inactive states. (f,g) H-bonds involving polar sidechains in helix 4 during trajectories describing a full transition between active and inactive states via transition states with a nearly intact helix 4 (f) and with a partially unfolded helix 4 (g). H-bonds observed during the middle segment of the transition are shown as triangles, while H-bonds present in the two stable end states are represented as open circles. On the horizontal axis, we marked relevant amino acids including mutations, which resulted in an increase in the activation barrier without affecting I and A13. Y101 can attain different orientations and its position is not strictly tied to the arrangement of T82 ( Supplementary Fig 3a,b ). This is in agreement with recent experimental data [25] ruling out the widely accepted Y-T coupling mechanism for activation. In sharp contrast, I (comprising the remaining 95% of the microstates) shows a surprising degree of variability, even in terms of the global arrangement and secondary structure content of helix 4. This macro-state also includes structures very close in secondary structure and backbone root mean squared distance (RMSD) to the active state model ( Fig. 2a , Supplementary Fig. 3c,d ). While the central section of helix 4 is well-defined in virtually all conformers, the two termini show a partial helical propensity as low as 20–30% ( Fig. 2f ). From the structural inspection of I, it is apparent that the tilt or register shift of helix 4 is not the fundamental feature distinguishing the two major conformers ( Fig. 2a ). Rather, the main difference separating the two ensembles is a change in helix α4 rotation around its axis associated with the rearrangement of specific sidechains, including Q96 and Y94 ( Fig. 2c,d,g,h ). The distributions of the rotational angle of helix α4 and the arrangement of Y94 with respect to helix α3 are distinct for the two macrostates, and these two order parameters are strongly correlated ( Fig. 2 ). Other order parameters do not distinguish the two macrostates, as shown, for example, by the bimodal distribution of F99 orientations ( Fig. 2e,i ). Interestingly, these results are consistent with both string calculations, which identify the change in the helix α4 rotation as a crucial coordinate capturing the important barrier separating I and A. Figure 2j shows a meta-trajectory constructed from the MSM visualizing a time trajectory of transitions ( Fig. 2j ). The result reinforces the findings that the rotation of helix 4 is the rate-limiting step for the inactive–active transition and that the calculated time scale is on the order of the experimentally measured transition rates ( Fig. 2j ) [12] . These time traces further illustrate the conformational heterogeneity of I on the low-microsecond time regime. Multiple pathways connect the two functional states Another feature suggested by our string pathway calculations is the possibility of substantially different pathways connecting the two end states. To explore this aspect and to capture some of the salient traits of the high-energy states crucial to the transition, we estimated microstate committor probabilities, based on the transition probability matrix of our MSM. Microstates with committor probabilities close to 0.5 provide detailed information about configurations close to the transition state ensemble. We find that the ensemble of microstates with committor probabilities close to 0.5 ( Fig. 3a ) is structurally diverse, in particular exhibiting a range of stabilities within helix 4 ( Fig. 3b,c ). Some of the ‘transition states’ have already attained a helical structure close to the end product, but with Y94 still trapped in the hydrophobic interface between helix α4 and strand β5 ( Fig. 3b ), while others have helix 4 partially unwound with only the central helix turn remaining intact ( Fig. 3c ). Figure 3: Multiple pathways connect the inactive and active states. ( a ) Committor probabilities for each of the 2,168 microstates in the MSM, defining the 5 most populated microstates belonging to the inactive and active macrostates as reactant and products, respectively. ( b , c ) Superposition of states with committor probabilities close to 0.5 indicates qualitative differences, ranging from an intact helix 4 ( b ) to a partially unfolded helix 4 ( c ). ( d , e ) Helical content and rotation angle of helix 4 during trajectories describing a full transition between active and inactive states. ( f , g ) H-bonds involving polar sidechains in helix 4 during trajectories describing a full transition between active and inactive states via transition states with a nearly intact helix 4 ( f ) and with a partially unfolded helix 4 ( g ). H-bonds observed during the middle segment of the transition are shown as triangles, while H-bonds present in the two stable end states are represented as open circles. On the horizontal axis, we marked relevant amino acids including mutations, which resulted in an increase in the activation barrier without affecting I and A [13] . Full size image Interestingly, some of the original MD trajectories initiated from the high energy starting structures, extracted from the middle of the string pathways, fully committed to the active or inactive macrostates. These trajectories constitute realistic unbiased pathways connecting the two functional states, thereby directly visualizing the activation mechanism at atomic resolution ( Fig. 3d,e ). To allow for the rotation around the helical axis and the concurring rearrangement of sidechains, the backbone of helix 4 undergoes a local destabilization to a different extent in different pathways. Consistent with the committor analysis, in some pathways only one turn at a time in helix 4 is disrupted, with the structures rapidly hopping among sub-states until the helix is fully stable and sidechains have reached a proper orientation ( Fig. 3d ). In other trajectories, the helix undergoes a more dramatic transition, with multiple helix turns lost simultaneously for short periods ( Fig. 3e ). The latter pathway is reminiscent of the ‘cracking’ model previously described for conformational transitions [17] . However, below we report on a crucial energetic feature connected to the ‘cracking’ that to our knowledge has not been found before. Nonnative H-bonds with multiple partners during transition An important common trait in the different transitions is the role of nonnative hydrogen bonds between sidechains, which are absent in the structures belonging to the I and A ground states ( Fig. 3f,g ). These transient H-bonds deliver an enthalpic stabilization of the structures during the transition. These findings agree with previous experiments, in which removal of several H-bond donors or acceptors for these nonnative H-bonds resulted in an increase in the activation barrier without affecting I and A [13] . Contrary to previous interpretations, however, these transient interactions appear to involve a number of partners, not just a single specific one: During a single trajectory, each of the sidechains can engage in direct interactions with a number of different partners, including interactions with backbone polar moieties that have temporarily lost their helical i—i+4 H-bond interactions ( Fig. 3f,g ). Many more interaction partners are observed in trajectories in which the helix undergoes more temporary unwinding, or cracking ( Fig. 3c,e,g ). Arguably, the crucial ingredient that facilitates the transition is precisely the presence of this group of polar sidechains that can assist and accompany the transition by variable nonnative interactions in strategic locations in the structure. This allows for efficient interconversion even when several stabilizing backbone i—i+4 interactions are temporarily lost. The fact that these interactions are not specific is compatible with the experimental observation that different H-bond-abolishing mutations had similar effects on the transition rates [13] . The degeneracy of these nonnative H-bonds provides an additional entropic advantage. The fact that in the original TMD simulations these interactions appeared to involve specific partners may result from the targeting bias. Our new results highlight the power and usefulness of unbiased all-atom methods such as MSMs. Direct sampling of transitions in long unbiased simulations The results from the MSM analysis suggest that transitions among conformers within I could be sampled directly in the course of several microseconds of simulation, and a chance to possibly even obtain a transition between A and I. We therefore performed two long, unbiased MD simulations ( ∼ 21 μs) starting from the inactive and active states shown in Fig. 1a on the special purpose machine ANTON [39] . The active state trajectory was extended to about 71 μs ( Supplementary Fig. 4 and ref. 25 ). These ANTON runs allow for a rigorous unbiased and independent study of conformational sampling of NtrC, and test if the MSM results were affected by the fact that the simulations were initiated from configurations extracted from the string pathway. The simulation initiated from A shows that the overall arrangement of α4 is remarkably stable. Some segments, particularly in the N-terminal region of α3 and α4 display some flexibility ( Fig. 4a , Supplementary Fig. 4 ). No transitions to the inactive states are observed, even when extending the simulation to ∼ 71 μs. Towards the end of the extended simulation, a few attempts to build the extra turn at the N terminus of α4 are observed ( Supplementary Fig. 4c ), but those are merely short-lived excursions into high-energy states that do not result in transitions to I. 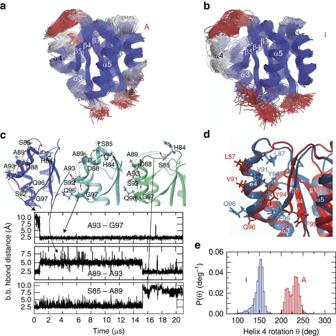Figure 4: Conformational sampling within the inactive and active states by long unbiased MD. Overlay of structures sampled during 21-μs unbiased MD simulations initiated from the active (a) and inactive (b) models. The structures are coloured from blue via grey to red according to the root mean squared fluctuations. (c) Conformers with substantial differences in the α4 helical arrangement are sampled during the inactive state simulation. The changes in several i, i+4 backbone H-bonds in α4 during the MD run are depicted. (d) Overlay of structures sampled respectively from the inactive state simulation (blue) and from the active state simulation (red). The secondary structure is almost overlapping; however, a crucial rotation of the α4 helix around its axis between the inactive and active conformer is observed, indicated by the arrangement of sidechains. (e) The simulations starting from the inactive and active state sample distinct distributions of α4 helix orientations. Figure 4: Conformational sampling within the inactive and active states by long unbiased MD. Overlay of structures sampled during 21-μs unbiased MD simulations initiated from the active ( a ) and inactive ( b ) models. The structures are coloured from blue via grey to red according to the root mean squared fluctuations. ( c ) Conformers with substantial differences in the α4 helical arrangement are sampled during the inactive state simulation. The changes in several i, i+4 backbone H-bonds in α4 during the MD run are depicted. ( d ) Overlay of structures sampled respectively from the inactive state simulation (blue) and from the active state simulation (red). The secondary structure is almost overlapping; however, a crucial rotation of the α4 helix around its axis between the inactive and active conformer is observed, indicated by the arrangement of sidechains. ( e ) The simulations starting from the inactive and active state sample distinct distributions of α4 helix orientations. Full size image In contrast, in the simulation initiated from I, the protein undergoes substantial rearrangements in the secondary structure of α4 and in the relative orientation of the helix’s axis with respect to the protein core. The helix position changes as a consequence of H-bond making/breaking events propagated from the C to the N terminus of helix 4 ( Fig. 4c ). During the simulation, however, the helix remains generally stable and does not undergo any unfolding events. This suggests that the protein is not merely undergoing a partial conformational transition visiting high-energy states, but is sampling an ensemble of states, all of which correspond to I. This finding together with the fact that snapshots extracted from the active and inactive simulations can have backbone r.m.s.d.’s as close as 2.5 Å ( Fig. 4d ) is fully consistent with the MSM analysis ( Supplementary Fig. 3 ). Furthermore, the position of sidechains in α4 linked to different helical rotation, the two order parameters identified by the MSM analysis that separate I and A, also distinguish both states in the Anton runs ( Fig. 4e ). This much slower transition to the other macro-state does not happen in either long simulation of the inactive or active starting conformation. NMR experiments support the free energy landscape model The computational results provide a novel perspective on the NtrC R activation process. While the description of the activation mechanism as a two-state model suggested in previous studies appears still valid in kinetic terms and in agreement with the NMR dynamics data [13] , the structural representation of the states needs to be revisited. The new model predicts that, while A is defined by a stable conformation of α4, I is comprised by a collection of conformers with diverse arrangements of α4, with variability in the average helical propensity in the termini ( Fig. 2f ). In particular, I is predicted to have at least partial helical propensity in the full region spanning H84 to Q96. Also, according to the new model, a clear signature distinguishing the two states would be different interactions of some of the amino acids sidechains reporting on the different angle of rotation of helix α4. For example, the sidechain of Y94 is close to helix 3 only in I, while Q96 is only close to helix 3 in A. To challenge our new computational model and provide an experimental test of these crucial hallmarks characterizing the two states, we performed new NMR experiments on both unphosphorylated and BeF 3 − -activated NtrC R . In previous NMR experiments on NtrC R recorded at 25 °C [11] , [12] , [13] , [14] , exchange broadening due to dynamics, exchange with water and the intrinsically lower sensitivity of older spectrometers hampered complete assignments and reduced the sensitivity in nuclear Överhauser enhancement spectroscopy (NOESY) signals. Particularly in the region around α3 and α4, only sparse distance information could be obtained. Advances in the spectrometers due to higher magnetic fields and a big increase in sensitivity by cryo probes, together with data acquisition at higher temperatures (35 °C), vastly improved the quality of our new NMR spectra. Besides full backbone assignments and almost complete side-chain assignments, significantly more NOE constraints were obtained. New structures for the inactive and active states were determined ( Fig. 5a,b ; Table 1 ). 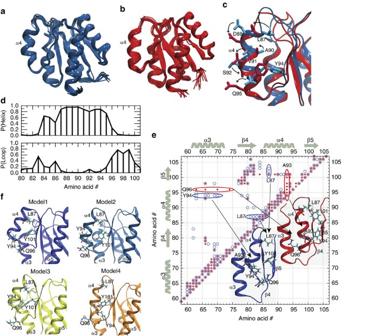Figure 5: New NMR structures buttress computational results. Structural models for apo (a) (2MSL) and BeF3−-activated form (b) (2MSK) from the refinement of the new NMR data sets. (c) An overlay of the two new structures shows a less pronounced difference in the global α4 helical arrangement relative to the previously available models. (d)Helical and loop propensity computed for each amino acid in the region of α4 using the chemical shifts of the apo protein. The helical propensity extends further in the sequence with respect to the previous available models for the nonphosphorylated form. (e) Representation of the NOE patterns in the apo (blue) and BeF3−-activated form (red) in the region of structural difference. Marked cross-peaks represent a NOESY peak between the corresponding amino acids. Distinct NOE patterns for the inactive (blue open circles) and active (red dots) states are circled and visualized on the corresponding structures. More specifically, a blue circle (red dot) in position I, J shows that in the NOESY spectra of the apo (BeF3−activated) form there is a NOE between atoms of amino acid I and atoms of amino acid J. (f) NMR models of nonphosphorylated NtrCRrelaxed in 50 ns MD simulations reproduce some of the variability we have observed in the other computational experiments. Figure 5: New NMR structures buttress computational results. Structural models for apo ( a ) (2MSL) and BeF 3 − -activated form ( b ) (2MSK) from the refinement of the new NMR data sets. ( c ) An overlay of the two new structures shows a less pronounced difference in the global α4 helical arrangement relative to the previously available models. ( d) Helical and loop propensity computed for each amino acid in the region of α4 using the chemical shifts of the apo protein. The helical propensity extends further in the sequence with respect to the previous available models for the nonphosphorylated form. ( e ) Representation of the NOE patterns in the apo (blue) and BeF 3 − -activated form (red) in the region of structural difference. Marked cross-peaks represent a NOESY peak between the corresponding amino acids. Distinct NOE patterns for the inactive (blue open circles) and active (red dots) states are circled and visualized on the corresponding structures. More specifically, a blue circle (red dot) in position I, J shows that in the NOESY spectra of the apo (BeF 3 − activated) form there is a NOE between atoms of amino acid I and atoms of amino acid J. ( f ) NMR models of nonphosphorylated NtrC R relaxed in 50 ns MD simulations reproduce some of the variability we have observed in the other computational experiments. Full size image Table 1 NMR refinement statistics. Full size table The new NMR model for the BeF 3 − -activated form is in full agreement with the active state model used in our calculations ( Fig. 5b , Supplementary Fig. 5 ). However, the structural description of the inactive state is significantly different from previous models ( Fig. 5a ). Since the new features describe important aspects of the inactive state ensemble and show striking agreement with the predictions from our MD simulations, we describe these in more detail: helix α4 is completely defined in the central region, while the two termini are only partially formed. This feature is confirmed by the helical propensity estimated from chemical shift values [40] ( Fig. 5d ). α4 partially extends up to Q96, whereas in the previous inactive model ( Fig.1 ) it ended at Y94 due to the fact that the signal coverage for Y94 to Q96 was scarce in the old data [14] . The extension of helix 4 is qualitatively consistent with our computational model, although the helical propensity measured by NMR is a little higher in both termini than predicted by the simulations ( Fig. 2f ). This might be partially due to the fact that in the NMR experiment of the apo protein, about 15% of the active state is sampled [12] , [13] , but may also indicate that our estimate of the relative populations of the sub-states constituting the inactive macrostate in our MSM analysis is not extremely accurate. The new NMR ensemble of the inactive state was further equilibrated in MD runs, gradually releasing the NMR restraints to better compare the experimental models with computation. Different MD runs diverge from the initial tight structural ensemble to different conformations, displaying some of the heterogeneity that was already observed in the MSM analysis ( Fig.5f , Supplementary Fig. 5 ). Importantly, despite the structural heterogeneity, the rotation of helix 4 around its axis is distinct between I and A ( Fig. 5c ), consistent with its identification from the MSM analysis as the key order parameter distinguishing both states. To further experimentally assess the relevance of the angle of rotation of helix 4 in defining the two states, we have scrutinized the NOESY peaks looking for signals confirming (or disproving) the exclusive interactions between residues in helix 4 and helix 3 predicted by our computational model. Consistent with our predictions, Y94 and Q96 indeed switch their relative positions with respect to helix 3 in the two states ( Fig. 5e ). In fact, while a series of NOESY peaks between Y94 and α3 are present in the data set of apo-NtrC R , these peaks disappear and signals between Q96 and helix 3 are detected for the BeF 3 − -activated form instead ( Fig. 5e ). In conclusion, the new NMR data fully support our new model that the change in the angle of rotation of helix α4 leading to the solvent exposure of different amino acid side chains is the slow degree of freedom that distinguishes I and A, and that I displays an intrinsic structural heterogeneity. One valuable, new structural information needs to be mentioned. Contrary to the previous structural models, the sidechain of F99 does not change position between the two states ( Supplementary Fig. 5b ). This might compromise some details regarding the rearrangement of the loop connecting α4 and β5 in our string calculations (mainly for Str1). Our modified structural NMR model for I could raise concern about the validity of the presented computer simulations. However, for the following reasons we are confident that the MSM analysis correctly describes the essential features for the free energy landscape. First, the unbiased MD runs for the MSM analysis were started from the string Str2, which originated from an accurate active state, and the F99 flip happened only at the very end of the transition ( Fig. 1i ). Therefore, the string calculations resulted in sampling almost all snapshots using accurate starting structures, including the correct F99 position seen in the new NMR structures. Consequently, most unbiased MD runs used in our MSM analysis sampled the proper F99 orientation. Second, our MSM analysis showed that switching of the F99 position does not constitute a crucial rate-limiting process ( Fig. 2e,i ). For these reasons, we conclude that this particular detail, although possibly affecting some detailed quantitative aspects of the relative populations of the sub-states belonging to the inactive state, does not affect the essence of our results about the pathways of interconversion. It is worth noting the very good agreement between the computational predictions and the new NMR experiments. Paradoxically, our computational results created an alert to question the accuracy of the original NMR models. A careful check of all NOESY assignments and structure calculations of the original data [12] , [14] reassured the accuracy of every procedure. However, the new and improved NMR spectra confirmed a new description of the inactive state, calling out a general warning sign that slightly incorrect structures can be obtained with fully coherent analysis when data are too sparse. Comparison of MSM models started from string and end states We now compare the results of our MSM analysis of the trajectories initiated from conformers along the pathway, performed with the Charmm27 (ref. 41 ) force field, with an independent MSM from simulations started from the two end states by the Pande lab [42] using Amber99SB (ref. 43 ). The major findings from the two calculations qualitatively agree, including the kinetic state definition of I and A, the time scale of I/A interconversion, their connection via multiple pathways and the crucial order parameter of helix 4 rotation that differentiates I from A ( Fig. 6a,b ). This overall agreement is a vital result because it demonstrates the robustness of the MSM method for characterizing conformational transitions crucial for biological function. 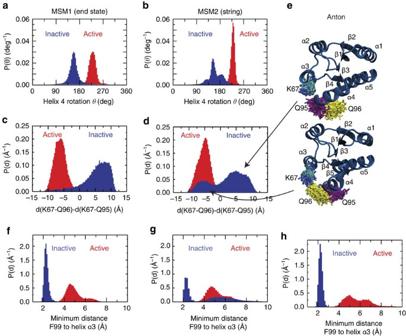Figure 6: Comparison between different MSM analyses. The distributions of some relevant order parameters highlight similarities and differences between the results presented by Vanattaet al.42(MSM1), obtained by simulation initiated from the active and inactive end states using the force field Amber99SB, and that of the present study (MSM2) obtained by simulations initiated from structures along the string pathway Str2 (seeFig. 1) using the force field Charmm27. (a,b) The rotation of helix 4 around its axis can separate active and inactive states in both studies. (c–e) The distribution of the distance between K67 and the glutamine residues Q95 and Q96 highlights the larger degree of heterogeneity of I observed in MSM2 (d), with respect to MSM1 (c). The same heterogeneity for the Q95/Q96 orientation is observed in unbiased inactive states simulations performed on Anton, shown by structural snapshots (e). (f–h) Position of F99 relative to helix3 for MSM1 (f), MSM 2 (g) and from the Anton run (h). Figure 6: Comparison between different MSM analyses. The distributions of some relevant order parameters highlight similarities and differences between the results presented by Vanatta et al. [42] (MSM1), obtained by simulation initiated from the active and inactive end states using the force field Amber99SB, and that of the present study (MSM2) obtained by simulations initiated from structures along the string pathway Str2 (see Fig. 1 ) using the force field Charmm27. ( a , b ) The rotation of helix 4 around its axis can separate active and inactive states in both studies. ( c – e ) The distribution of the distance between K67 and the glutamine residues Q95 and Q96 highlights the larger degree of heterogeneity of I observed in MSM2 ( d ), with respect to MSM1 ( c ). The same heterogeneity for the Q95/Q96 orientation is observed in unbiased inactive states simulations performed on Anton, shown by structural snapshots ( e ). ( f – h ) Position of F99 relative to helix3 for MSM1 ( f ), MSM 2 ( g ) and from the Anton run ( h ). Full size image We also find differences in the two studies, which point to significant differences in currently used force fields in agreement with other studies [44] , but also to a potential advantage of using a string as starting point for a MSM analysis. In our string-based MSM, we see a larger structural heterogeneity of I as illustrated by the probability distribution of the distances of Q96 and Q95 to K67 ( Fig. 6c,d ). This heterogeneity results from conformational sampling within I, reaching up to 10 μs, which is at least 1 order of magnitude slower compared with the relaxation processes found by Vanatta et al. [42] Our ANTON runs identify different force fields (Amber99SB in the MSM of ref. 42 versus Charmm27 in our MSM and ANTON runs) as the source of this increased heterogeneity, because they reveal the same heterogeneity and time scale of sampling within inactive state found by our MSM. Note that the ANTON run was started from the same starting structure as in the study by Vanatta et al. [42] . The F99-switch identified in the MSM analysis of Vanatta seems to result from the incorrect F99 position in the initial NMR structure, which was overcome in our MSM analysis by the use of the string method prior to the MSM as explained above. This observed difference is not due to different force fields because in our ANTON runs the inactive ensemble F99 is also trapped in the original wrong configuration ( Fig. 6f–h ). In addition, we find (i) a larger number of configurations with committor probabilities around 0.5, (ii) pathways with significantly different transition states and (iii) nonnative H-bonds with multiple partners during the transition in our MSM analysis. The increased structural heterogeneity of our MSM likely results from initializing the MD runs from the diverse, high free energy configurations obtained from the string pathway. Our findings are substantiated by the direct detection of full interconversion between I and A in single unbiased MD runs. Current design of protein function is largely based on the successful prediction of protein structures [2] , [3] . The superior performance of naturally evolved enzymes compared with current designs is thought to be primarily rooted in nature’s fine-tuned ability to efficiently sample conformational substates [45] . While this dynamic nature has generally been acknowledged to be crucial for biomolecular function, our current understanding is in its infancy. Here we characterize the free energy landscape of the inactive/active interconversion in a signalling protein with an atomic lens, to uncover novel and potentially general features nature evolved for specific and efficient signaling. A combination of the string method, MSM analysis and long MD runs on ANTON delivered a coherent new structural view of the two functional states, and provided new insight into the transition pathways connecting the states: First, while the active state features a narrow structural ensemble, the inactive state consists of conformers that are structurally as different among each other as from the active state. These sub-states can interconvert on timescales of the order of a few microseconds, while the transition to the active state occurs in about 100 μs. The different nature of the two functional states is compelling in light of evolutionary pressure for function. While a defined active conformation is needed to guarantee a specific interaction with the downstream partner, switching off the signalling cascade can be accomplished by any conformation other than the active structure. The intrinsic entropic nature of the inactive state may not be a limitation in the efficiency of the conformational transition, but rather provides an advantage. Second, we find multiple pathways connecting the two states with quite different transition states. The similarity of this finding to protein folding pathways [27] , [28] , [29] , [30] is intriguing, and has been observed in computational studies of other native state dynamics [6] , [10] , [46] , [47] . Multiple pathways overcome the extreme ‘bottleneck’ problem resulting in a higher probability of the activation process, resulting in lowering the entropic barrier of conformational transitions. Last, a detailed analysis of the pathways exposed atomistic details of enthalpic contributions to the lowering of the transition energy barrier. During the transition, a number of transient interactions involving polar sidechains, strategically positioned in the sequence, enthalpically compensate for some of the energetic penalties from the temporary loss of backbone H-bonds. While we previously hypothesized that specific nonnative H-bonds are responsible for lowering the activation barrier [13] , we now learn that nature ‘designed’ these nonnative interactions to be more widely distributed, with several possible partners during the transition, making the whole system more robust. These findings amplify the sophistication of naturally evolved functional proteins, relative to the current understanding and consequently the implementation of current design strategies. Again, we want to highlight the striking analogy to the role of nonnative contacts during protein folding [28] . Despite a number of studies reported for NtrC R (refs 16 , 17 , 18 , 19 , 20 , 21 , 22 , 23 ), these novel and critical principles of the free energy landscape have been missed in the past. Our results illustrate the need of unbiased and reaction coordinate-free MD methods for exploring the free energy landscape of complex conformational transitions within the native state. Our new findings of a degenerate inactive state ensemble, its connection to multiple transition pathways within the native state and finally the clever usage of a series of nonnative contacts to facilitate biologically essential transitions while avoiding unfolding, may be general features for dynamic processes in other native proteins, including enzyme catalysis and other biological functions. Pathway calculations The procedure for obtaining the minimum free energy pathway was implemented as proposed by Pan et al. [18] . The method consists of an iterative procedure in which an initial pathway, discretized as an ordered chain of states (called images in this context) is represented as a curve (‘string’) in a multidimensional space of collective variables and progressively relaxed to the local minimum free energy pathway. At each iteration three steps are performed: First each image is restrained to the vicinity of the corresponding point in the collective variable space and configurations compatible with the appropriate values of the collective coordinates are harvested during a restrained MD simulation. Then, for each image, a series of short unbiased MD are started from the configurations harvested during the restrained simulations. The average drift along the free energy gradients is measured. Finally, the position of the images is updated by first moving the points in the direction of the measured gradients, and then redistributing them to maintain a uniform spacing along the pathway, following the strategy proposed by Maragliano et al. [48] . The value of the r.m.s.d. in the collective variable space between the current state of the string and the initial reference pathway is used to judge the convergence of the iterative procedure ( Supplementary Fig. 1 ). Here follow details on the generation of the input pathways and implementation of the iterative procedure for the two pathways Str1 and Str2: The input pathway for the string Str1 was obtained by extracting 26 protein configurations distributed along the TMD trajectory described by Lei et al. [22] with a few changes based on new NMR data and computational results. The resulting configurations were parametrized with the CHARM27 force field [41] including the CMAP correction and solvated with 7366 TIP3P water molecules in a rhombic dodecahedron unit cell. The charge of the system was neutralized with sodium ions. Periodic boundary conditions were applied to the simulation cell. The solvated structures were minimized with the conjugate gradient method as implemented in NAMD [49] , and then gradually heated to 300 K with a time step of 1 fs while keeping positional restraints on all heavy atoms. Electrostatics was treated with the Particle Mesh Ewald scheme [50] . The bonds of all hydrogen atoms were constrained with the SHAKE algorithm [51] . During the pathway optimization, 190 distances between heavy atoms in the region of helix α4 were used as collective variables. The iterative string optimization procedure was implemented as follows: For each image, a restrained 50 ps NPT simulation (constant number of particles N, constant pressure P =1.01325 bar, constant temperature T =300 K), was performed using the software NAMD. The temperature was controlled with the Langevin dynamics method, while keeping the pressure constant using the combined Langevin piston Nose–Hoover method [52] . Electrostatics was computed using particle mesh ewald (PME) with a grid with 72 points in each dimension. The time step for the integration was set to 1 fs. Restraints in the collective variables space were implemented using the NAMD ‘colvars’ module. For each of the 100 configurations harvested in the restrained simulation, a 3 ps unbiased simulation was performed. The same simulation parameters as in the restrained simulation were used. The restraints were turned off and the time step was increased to 2 fs. For the generation of the Str2 pathway, the two end structures of the TMD of Lei et al. [22] were equilibrated, after being patched according to new NMR data and computational results. The A and I structures were minimized with a series of conjugate gradients minimizations, and equilibrated in NVT ensemble raising the temperature from 50 to 300 K, in steps of 25 K while gradually releasing constraints from the protein. Each temperature interval was simulated for 50 ps. Hydrogen atoms were constrained with SHAKE [51] . During the NVT equilibration, the time step was set to 1 fs. After reaching 300 K, the density of the system was equilibrated during a NPT ( T =300 K, P =1.01325, bar) run. Electrostatics was computed with PME, with a grid with 72 points in each dimension. Non-bonded interactions were gradually switched to 0 between 12 and 14 Å during heating and between 10 and 12 Å during the NPT. The temperature was controlled with the Langevin dynamics method, while keeping the pressure constant using the combined Langevin piston Nose–Hoover method [52] . The structures obtained after 50 ns of equilibrations were then used to generate a new TMD pathway connecting the active and inactive conformer. The starting point of the TMD simulation was the active conformation. The r.m.s.d. to the inactive structure was reduced to a target value of 0.5 Å in a 6 ns simulation with a force constant of 200 kcal mol −1 Å −2 . From the resulting trajectory, 80 frames were extracted and used as input pathway for the string optimization procedure. During the pathway optimization, 210 distances between heavy atoms in the region of helix α4 were used as collective variables. The iterative string optimization procedure was implemented as follows: for each image, a 50 ps NVT simulation ( T =300 K) was performed using the software GROMACS [53] . The temperature was controlled with a V-rescale temperature coupling as implemented in GROMACS. Electrostatics was computed using the PME method with a grid size of 1 Å. The time step for the integration was set to 2 fs. Van der Waals interactions were switched off between 10 and 12 Å. Restraints in the collective variable space were implemented using the PLUMED software [54] . For each of the 100 configurations harvested in the restrained simulation, a 5 ps unbiased run was performed. The same simulation parameters as in the restrained simulation were used. The restrained were turned off. To estimate the free energy profile along the pathway, umbrella sampling simulations were performed using as a reaction coordinate the progression along a piecewise linear approximation of string arc-length connecting the images. In each of the segments connecting 2 subsequent images along the converged pathway, 20 simulations were performed sampling values of the projection of the position in the collective variable space onto the vector connecting the 2 images. A total of 500 simulations were performed for Str1 (total of ∼ 414 ns) and 1,579 for Str2 (total of 1,446 ns). The sampled distributions were then used to reconstruct the free energy profile with a weighted histogram analysis procedure [55] , [56] ( http://membrane.urmc.rochester.edu/content/wham/ ). To estimate the error on the reconstructed profiles, the weighted histogram analysis was repeated 10 times, discarding 10–20% of the data each time. Markov state model The 80 images of the optimized pathway Str2 were used as starting conformations for 8,000 independent simulations, 100 per each image, initiated with different initial velocities drawn from a Maxwell–Boltzmann distribution at 300 K. The simulations were run on the Folding@Home distributed computing infrastructure [35] . The simulations were performed in the NVT ensemble, using a Nose–Hoover thermostat to keep the temperature at 300 K. Electrostatics was treated with PME, with a grid spacing of 1.2 Å. The Van der Waals interactions were switched off between 9 and 10 Å. The short-range electrostatic interactions had a real space cutoff of 12 Å. The neighbour list was grid based and updated every 20 fs with a cutoff of 12 Å. Bonds were constrained using the LINCS algorithm. The time step was 2 fs. Configurations were saved every 10 ps. During the data harvesting a total of 1.015 ms simulation time was collected. The distribution of the lengths of the individual trajectories is shown in Supplementary Fig. 2 . In the MSM analysis, we have preprocessed the trajectories, removing from the data set trajectories shorter than 15 ns, leaving a total of about 978 μs. We have also subsampled the trajectories maintaining configurations every 0.2 ns. The MSM analysis (see for example, [37] , [57] and references therein) was performed using the software MSMbuilder [58] . In the initial state of the analysis, the configurations were clustered structurally using a mixed K-centre–K-medoids algorithm. In a first step, a K-centre clustering is performed, followed then by 10 iterations of K-medoids. To make the clustering problem more tractable, we used only one configuration every 5 ns. When comparing 2 configurations, the pairwise distance used was the r.m.s.d. among backbone and Cβ atoms of the amino acids in the region 82–101, after the 2 configurations were aligned using the backbone atoms of the remaining part of the structure. The cutoff used in the K-medoids step was 2 Å. The clustering resulted in 2,168 microstates. After having identified the cluster centres, the remaining configurations were assigned to the closest cluster and used to build a transition probability matrix among the microstates, by counting the transitions between the states. The calculation was repeated at different lagtimes Δ t , obtaining an analysis of the implied relaxation timescales as function of Δ t ( Supplementary Fig S2 ). Convergence of the implied timescales is obtained for a lagtime of 50 ns. The transition probability matrix corresponding to Δ t =50 ns is used in the analysis. The transition probability matrix was then used as a basis for lumping states in 2 or 10 macrostates using the PCCA method [36] , [38] as implemented in MSMbuilder [58] . The ability of the macrostate model to recapitulate the kinetic observed in the raw MD data is assessed with a Kolmogorov–Chapman test [33] ( Supplementary Fig. S2 ). Long unbiased simulations on Anton The equilibrated structures of A and I conformations used as end states for initiating the string calculation Str2, were used as starting points for test and production runs performed on the supercomputer Anton [39] , designed by DESRES research and made available to us through a NIH funded programme at Pittsburgh Supercomputing Center. After being further equilibrated in a rectangular box at 320 K, the configurations for A and I were prepared to run on Anton using a set of scripts provided by the staff at PSC. For the production runs, we used a time step of 2.5, a 32 × 32 × 32 fast Fourier transform (FFT) mesh and a 1:1:2 reference system propagation algorithm (RESPA) scheme. With those parameters, the energy drift rate in test NVE simulations was ∼ 0.017 kcal mol −1 per degree-of-freedom (dof) per μs, which matches DESRES results for systems of similar size [39] . The system was simulated in NVT ensemble, coupled to a Nose–Hoover thermostat at 320 K. The simulations of the active and inactive models were initially performed for ∼ 21 μs. As described in a separate study [25] the simulation of the active state was extended to a total of ∼ 71 μs to enable a detailed investigation of the role of Y101 and T82 in the activation process. In Fig. 3 of the main text only analysis from the initial 21 μs of the active state simulation is presented, to allow a more direct comparison with the inactive state simulation of the same length. In Supplementary Fig. 4 the analysis presented comprises the full 71 μs available data of the active state simulation. NMR structure refinement Isotopically labelled apo- and BeF 3 − -labelled NtrC R were prepared as previously described [12] . NMR experiments for assignment and measurement of J-couplings were performed in a Varian INOVA 600 MHz spectrometer with a gradient-equipped room-temperature triple-resonance probe. NOESY spectra were obtained from a Bruker Avance II 800 MHz spectrometer with a TCI cryoprobe. All spectra were obtained at 35 °C. Processing was performed using NMRPipe [59] . J-coupling spectra were analysed using NMRViewJ [60] . Resonance and NOE assignments were performed using CARA ( http://cara.nmr.ch ). Assignments of apo- and BeF 3 − NTRC R were collated using HNCO, HNCACB, CBCA(CO)NH [61] triple-resonance spectra. Sidechains were assigned using (H)C(CO)NNH-, H(CCO)NNH- [62] , HCCH- [63] and HCCH 3 -TOCSY [64] spectra. Aromatic side chains were assigned using (HB)CB(CGCD)HD and (HB)CB(CGCDCE)HE [65] spectra and NOESYs. Assignments were 98% complete. Distance restraints were determined using NOESY-15N-HSQC spectra, as well as two NOESY-13C-HSQC spectra centred on the aliphatic and aromatic regions. Backbone dihedral angle restraints were calculated using TALOS+ [66] . Side-chain dihedral angles were restrained using J-couplings calculated from spin-echo-difference spectra for J CO–Cγ and J N–Cγ of methyl-bearing [67] and aromatic [68] residues. Additional side-chain dihedral angle restraints were calculated from chemical shifts. Structure calculations were performed using CYANA [69] . Initially, unassigned NOESY peak lists were given to the programme and automatically assigned as part of the minimization process. The resulting distance restraints, along with predicted contacts of <4 Å, were then manually checked against the actual spectra. Manually verified distance restraints and angular restraints were then supplied to CYANA for final structure calculation. For the BeF 3 − -labelled protein, 638 long-range NOEs (1,866 total), 172 backbone angle restraints and 48 side-chain dihedral angle restraints were used. For apo-NtrC R , 984 long-range NOEs (2,282 total), 128 backbone angle restraints and 48 side-chain angle restraints were used. The 25 lowest energy conformers from each minimization were used in subsequent steps. The 10 lowest energy models of the apo-NtrC R obtained in the structural refinement with CYANA have been further equilibrated in MD simulation in explicit water, with the following protocol: The structures were first minimized via a series of conjugated gradients and then equilibrated in NVT ensemble increasing the temperature from 150 to 300 K, in steps of 50 K, gradually reducing the constraints on the protein atoms. Hydrogen atoms were constrained with SHAKE. During the NVT equilibration, the time step was set to 1 fs. After reaching 300 K, the density of the system was equilibrated during a 2 ns NPT ( T =300 K, P =1.01325, bar) run. The temperature was controlled with the Langevin dynamics method, while keeping the pressure constant using the combined Langevin piston Nose–Hoover method [52] . Long-range electrostatic interactions were treated with PME, with a grid spacing of 1 Å. Non-bonded cutoff was switched off from 12 to 14 Å during heating and from 10 to 12 Å during the NPT simulation. The equilibration of the models was then continued in GROMACS. The simulations were performed in the NPT ensemble, using a Nose–Hoover thermostat to keep the temperature at 300 K and the Parrinello–Rahman [70] coupling to target a reference pressure of 1 bar. The electrostatic was treated with PME, with a grid spacing of 1.2 Å. The Van der Waals interactions were switched off from 9 to 10 Å. The short-range electrostatic interactions had a real space cutoff of 12 Å. The neighbour list was grid based and updated every 20 fs with a cutoff of 12 Å. Bonds were constrained using the LINCS algorithm. The time step for the integration was 2 fs. During the first 10 ns of the simulations, distance restraints from the NOE analysis and backbone dihedral restraints obtained from the statistical-based analysis performed with TALOS were added to the simulation. After 10 ns, the restraints were switched off and each of the simulations was continued for additional 50 ns. Figures were produced using VMD ( http://www.ks.uiuc.edu/Research/vmd/ ), Grace ( http://plasma-gate.weizmann.ac.il/Grace/ ), Matplotlib ( http://matplotlib.org ) and Gnuplot ( http://www.gnuplot.info ). Accession codes: The coordinate and chemical shift data were deposited in Protein Data Bank under accession codes 2MSL (NtrC R inactive state) and 2MSK (NtrC R active state). How to cite this article: Pontiggia, F. et al. Free energy landscape of activation in a signalling protein at atomic resolution. Nat. Commun. 6:7284 doi: 10.1038/ncomms8284 (2015).